Disappearance of nodal gap across the insulator–superconductor transition in a copper-oxide superconductor The parent compound of the copper-oxide high-temperature superconductors is a Mott insulator. Superconductivity is realized by doping an appropriate amount of charge carriers. How a Mott insulator transforms into a superconductor is crucial in understanding the unusual physical properties of high-temperature superconductors and the superconductivity mechanism. Here we report high-resolution angle-resolved photoemission measurement on heavily underdoped Bi 2 Sr 2– x La x CuO 6+ δ system. The electronic structure of the lightly doped samples exhibit a number of characteristics: existence of an energy gap along the nodal direction, d -wave-like anisotropic energy gap along the underlying Fermi surface, and coexistence of a coherence peak and a broad hump in the photoemission spectra. Our results reveal a clear insulator–superconductor transition at a critical doping level of ~0.10 where the nodal energy gap approaches zero, the three-dimensional antiferromagnetic order disappears, and superconductivity starts to emerge. These observations clearly signal a close connection between the nodal gap, antiferromagnetism and superconductivity. The parent compound of the copper-oxide superconductors is an antiferromagnetic Mott insulator; doping of charge carriers into the parent compound leads to an insulator–metal transition and the emergence of high-temperature superconductivity (SC) [1] . In the superconducting state, predominantly d -wave superconducting gap is well established with a zero gap along the nodal direction [2] . In the normal state of the underdoped superconducting region, anisotropic pseudogap appears with a zero gap along the nodal direction [3] . A particular, yet important, region exists between the parent compound and the superconducting region, that is, a lightly doped region where, on slight doping, the three-dimensional (3D) antiferromagnetic order is rapidly suppressed and an insulator–metal transition occurs. What is the main reason for the antiferromagnetic phase remaining insulating after being doped? What are the electronic characteristics of this peculiar lightly doped region? How is the electronic structure of this particular region connected to the pseudogap and superconducting gap in the underdoped superconducting region? Investigation of this lightly doped region is critical in understanding how a Mott insulator can transform into a d -wave superconductor, the origin of the pseudogap and its relationship with the superconducting gap [4] , [5] . In this paper, we report angle-resolved photoemission (ARPES) measurements on the electronic structure evolution with doping in Bi 2 (Sr 2– x La x )CuO 6+ δ (La–Bi2201) system focusing on the lightly doped region and the insulator–superconductor transition. Our super-high-resolution ARPES experiments reveal an insulator–superconductor transition at a critical doping level of P ~0.10. In the lightly doped region ( P =0−0.10), the photoemission spectra are characterized by the coexistence of a coherence peak and a broad hump consistent with a polaronic behaviour. Moreover, a fully opened d -wave-like anisotropic energy gap is observed, which is offset by an energy gap along the (0,0)-( π,π ) nodal direction. The nodal gap decreases with increasing doping and approaches zero at a critical doping level of P ~0.10, where the 3D antiferromagnetic order vanishes and SC starts to emerge [6] . In addition, a smooth transition from the energy gap in the lightly doped region to the pseudogap in the underdoped superconducting region is observed. These observations indicate a close relationship between the nodal energy gap, antiferromagnetic insulating phase and SC. They will shed important light on the origin of the pseudogap in high-temperature superconductors, and point to the importance of combining the electron correlation, antiferromagnetism (AF) and strong electron–phonon coupling in understanding the electronic structure of the lightly doped and underdoped regions. 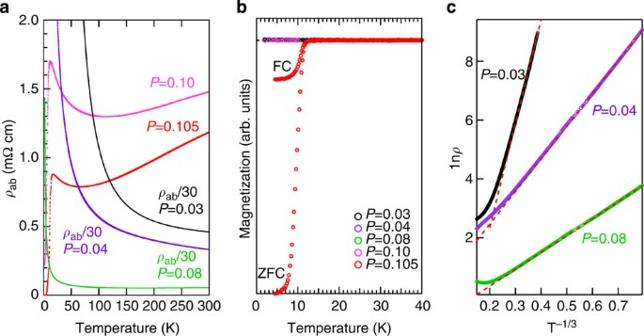Figure 1: Transport and magnetic measurements of the La–Bi2201 samples. (a) Temperature dependence of the in-plane resistivityρabof the La–Bi2201 single crystals. (b) Magnetization measurements of the La–Bi2201 single crystals with a magnetic field of 1 Oe. FC refers to the field-cooled measurement, whereas ZFC refers to zero field-cooled measurement. (c) The in-plane resistivity–temperature curves plotted as lnρ~T−1/3for the La–Bi2201 single crystals with low doping levels of 0.03 (black circles), 0.04 (violet circles) and 0.08 (green circles). The dashed red lines are linear that serve as a guide to the eyes. Over an extended range of low temperature, these curves show a linear dependence. Transport properties of La–Bi2201 Figure 1 shows the temperature dependence of the in-plane resistivity ρ ab ( Fig. 1a ) and the magnetization ( Fig. 1b ) of the La–Bi2201 single crystals. The La–Bi2201 samples with P =0–0.08 doping levels are non-superconducting. The P =0.10 sample is superconducting with a T c at ~3 K, which is on the border of insulator-to-superconductor transition. The P =0.105 sample has a T c of 12 K. Figure 1: Transport and magnetic measurements of the La–Bi2201 samples. ( a ) Temperature dependence of the in-plane resistivity ρ ab of the La–Bi2201 single crystals. ( b ) Magnetization measurements of the La–Bi2201 single crystals with a magnetic field of 1 Oe. FC refers to the field-cooled measurement, whereas ZFC refers to zero field-cooled measurement. ( c ) The in-plane resistivity–temperature curves plotted as ln ρ ~ T −1/3 for the La–Bi2201 single crystals with low doping levels of 0.03 (black circles), 0.04 (violet circles) and 0.08 (green circles). The dashed red lines are linear that serve as a guide to the eyes. Over an extended range of low temperature, these curves show a linear dependence. Full size image It is interesting to note that, the insulator–superconductor transition takes place near the universal two-dimensional (2D) resistance, h /4 e 2 , which corresponds to 3D resistivity ~0.8 mΩ·cm in Bi2201. The insulator–superconductor transition can also be driven by Zn doping [7] or by changing the thickness of cuprate thin films [4] , and it is known that it takes place at nearly the same resistance values. The in-plane resistivity–temperature curves of the La–Bi2201 single crystals with low doping levels of 0.03, 0.04 and 0.08 are re-plotted in Fig. 1c as ln ρ ~ T −1/3 . Over an extended range of low temperature, these curves show a linear dependence. This is consistent with the 2D variable-range hopping model, where the resistivity–temperature dependence is expected to be: ρ = ρ 0 e ( T 0 / T ) 1 / 3 (refs 8 , 9 ). 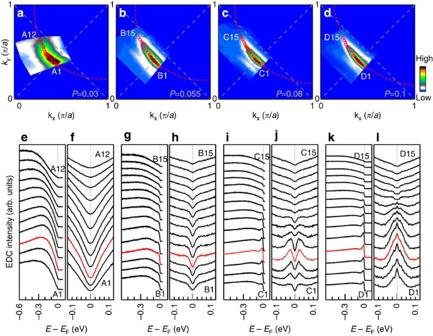Figure 2: Observation of the nodal gap in lightly doped La–Bi2201 samples. (a–d) The momentum distribution of the spectral weight integrated within a (−10 meV, 10 meV) energy window aroundEFfor La–Bi2201 samples with different doping levelsPof 0.03 (a), 0.055 (b), 0.08 (c) and 0.10 (d). The data were taken at a temperature of 20 K. The location of the ‘underlying Fermi surface’ is labelled by red empty circles and the red dashed lines are obtained by tight-binding fitting to the circles, which serve as a guide to the eyes. The photoemission spectra (energy distribution curves, EDCs) along the ‘underlying Fermi surface’ are shown in (e), (g), (i) and (k) for the doping levels of 0.03 (e), 0.055 (g), 0.08 (i) and 0.10 (k), respectively. The corresponding symmetrized EDCs are shown in (f), (h), (j) and (l). Red lines indicate the EDCs and symmetrized EDCs along the (0,0)-(π,π) nodal direction. We paid special attention to avoid any charging effect due to the insulating behaviours of these lightly doped samples. We varied the photon flux over a large range and observed little change in the measured EDCs. Underlying Fermi surface Figure 2 shows the doping evolution of the underlying Fermi surface across the non-superconductor–superconductor transition and indications of the nodal energy gap observed for the lightly doped La–Bi2201 samples. As seen from Fig. 2a–d , in the lightly doped samples, the spectral weight distribution dominates near the ( π /2, π /2) nodal region and then spreads towards the (0, π ) antinodal region with increasing doping. As commonly used before, we denote the high-intensity contour in the spectral weight distribution as the ‘underlying Fermi surface’, although in principle a strict Fermi surface refers to the locus of momentum without an energy gap [10] . The photoemission spectra (energy distribution curves, EDCs) along the underlying Fermi surface are displayed in Fig. 2e,g,i,k for different doping levels, with their corresponding symmetrized EDCs shown in Fig. 2f,h,j,l respectively. The EDC symmetrization is an empirical and intuitive way to examine the existence of an energy gap by removing the Fermi distribution function from the original ARPES data [11] . As seen from Fig. 2e , with very low doping of P =0.03, only a broad hump feature dominates the measured spectra. It disperses towards low binding energy, reaches its minimum ~200 meV along the nodal direction and then turns back. The spectral weight near the Fermi level E F is strongly suppressed for this lightly doped sample, and there is apparently a gap opening ( Fig. 2f ). Further increase of the doping to P =0.055 results in an emergence of a coherence peak near the Fermi level, which coexists with the broad hump structure ( Fig. 2g ). A close inspection reveals an energy gap for the coherence peak along the entire underlying Fermi surface, including the nodal region ( Fig. 2h ). When the doping level reaches P =0.08, the coherence peak becomes prominent. In the meantime, the broad hump gets weaker but remains visible ( Fig. 2i ). The energy gap opening is clear along the entire underlying Fermi surface ( Fig. 2j ). Eventually, when the doping level becomes P =0.10, the coherence peak gets sharp and the broad hump remains discernable ( Fig. 2k ). But in this case, no indication of an energy gap opening is observed near the nodal region ( Fig. 2l ). However, there are clear indications of gap opening in the EDCs far away from the nodal region. This is consistent with the observation of the Fermi arc in underdoped superconducting samples [12] , [13] , [14] . Figure 2: Observation of the nodal gap in lightly doped La–Bi2201 samples. ( a – d ) The momentum distribution of the spectral weight integrated within a (−10 meV, 10 meV) energy window around E F for La–Bi2201 samples with different doping levels P of 0.03 ( a ), 0.055 ( b ), 0.08 ( c ) and 0.10 ( d ). The data were taken at a temperature of 20 K. The location of the ‘underlying Fermi surface’ is labelled by red empty circles and the red dashed lines are obtained by tight-binding fitting to the circles, which serve as a guide to the eyes. The photoemission spectra (energy distribution curves, EDCs) along the ‘underlying Fermi surface’ are shown in ( e ), ( g ), ( i ) and ( k ) for the doping levels of 0.03 ( e ), 0.055 ( g ), 0.08 ( i ) and 0.10 ( k ), respectively. The corresponding symmetrized EDCs are shown in ( f ), ( h ), ( j ) and ( l ). Red lines indicate the EDCs and symmetrized EDCs along the (0,0)-( π , π ) nodal direction. We paid special attention to avoid any charging effect due to the insulating behaviours of these lightly doped samples. We varied the photon flux over a large range and observed little change in the measured EDCs. 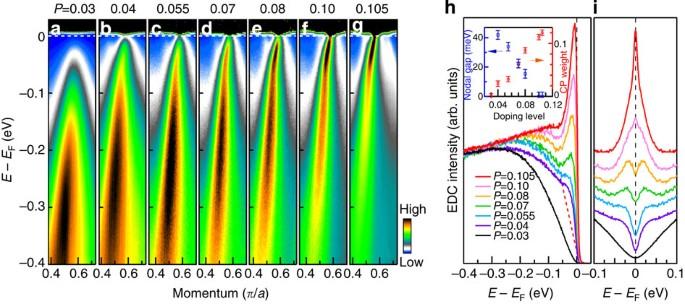Figure 3: Doping evolution of the nodal gap in lightly doped La–Bi2201 samples. (a–g) Band structures measured along the nodal direction for the La–Bi2201 samples with different doping levelsPof 0.03 (a), 0.04 (b), 0.055 (c), 0.07 (d), 0.08 (e), 0.10 (f) and 0.105 (g). The data were taken at a temperature of ~15 K and were divided by the Fermi distribution function to highlight the gap opening near the Fermi level. Panelhshows the original EDCs on the ‘underlying Fermi surface’ along the nodal direction; the corresponding symmetrized EDCs are shown ini. The top-left inset inhshows the doping dependence of the nodal gap (blue empty squares) and the coherence peak (CP) spectral weight (red empty circles). The nodal gap is obtained by taking the peak position of the symmetrized EDCs ini. The CP spectral weight (CP weight) is defined by the ratio between the peak area and the overall spectral weight integrated over the (−0.4 eV, 0.03 eV) energy window. The coherence peak area is obtained by subtracting a linear background (red dashed line) as illustrated inhfor the EDC of theP=0.04 sample. Full size image Nodal band structure Figure 3 focuses on the nodal gap and its detailed doping evolution. Figure 3a–g shows doping evolution of the band structure along the nodal direction. The Fermi distribution function is divided out from these data to facilitate the revelation of the energy gap near the Fermi level. Original EDCs for the La–Bi2201 samples with different doping levels are shown in Fig. 3h on the underlying Fermi surface along the nodal direction, with their corresponding symmetrized EDCs shown in Fig. 3i . From the raw data ( Fig. 3a–g) , it is clear that with increasing doping, the spectral weight transfers from high binding energy to low binding energy. For the P =0.03 sample, the spectral weight near E F is strongly depleted ( Fig. 3a ) and the nodal EDC is characterized by a prominent broad hump near 250 meV. A slight increase of the doping level to 0.04 brings a significant amount of spectral weight towards low binding energy and a weak coherence peak emerges near the Fermi level ( Fig. 3b,h ). Further doping brings more spectral weight to the Fermi level so that the coherence peak becomes sharper, while the broad hump structure becomes weaker. The relative spectral weight increase of the coherence peak with increasing doping is shown in the inset of Fig. 3h (red circles). A similar trend was observed before in other cuprates [15] , [16] . We note that, compared with the previous results [17] , [18] , this is the first time one can observe clear coherence peaks below the doping level of P =0.10 in Bi2201 and a coexistence of peak-dip-hump structure for such low doping samples. This is mainly due to sample quality improvement and the utilization of super-high-resolution of our laser-ARPES measurements. The observation of a clear coherence peak near the Fermi level makes it possible to precisely determine the energy gap. As shown in the symmetrized nodal EDCs in Fig. 3i , whereas the symmetrized EDC of the P =0.03 sample becomes featureless near E F , there is a clear indication of nodal gap opening in the samples with doping of P =0.04 to P =0.08. Such a nodal gap is closed for the P =0.10 and P =0.105 samples. As shown in the inset of Fig. 3h , the nodal gap drops monotonically with increasing doping until the doping level of 0.10, which just becomes superconducting with a T c ~3 K. Figure 3: Doping evolution of the nodal gap in lightly doped La–Bi2201 samples. ( a – g ) Band structures measured along the nodal direction for the La–Bi2201 samples with different doping levels P of 0.03 ( a ), 0.04 ( b ), 0.055 ( c ), 0.07 ( d ), 0.08 ( e ), 0.10 ( f ) and 0.105 ( g ). The data were taken at a temperature of ~15 K and were divided by the Fermi distribution function to highlight the gap opening near the Fermi level. Panel h shows the original EDCs on the ‘underlying Fermi surface’ along the nodal direction; the corresponding symmetrized EDCs are shown in i . The top-left inset in h shows the doping dependence of the nodal gap (blue empty squares) and the coherence peak (CP) spectral weight (red empty circles). The nodal gap is obtained by taking the peak position of the symmetrized EDCs in i . The CP spectral weight (CP weight) is defined by the ratio between the peak area and the overall spectral weight integrated over the (−0.4 eV, 0.03 eV) energy window. The coherence peak area is obtained by subtracting a linear background (red dashed line) as illustrated in h for the EDC of the P =0.04 sample. Full size image To understand the origin of the nodal gap in the lightly doped samples, it is important to investigate its temperature dependence. 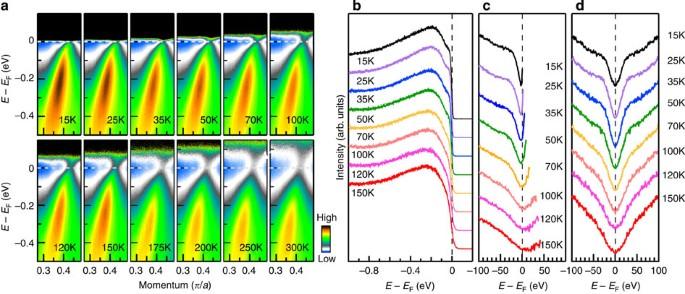Figure 4: Temperature dependence of the nodal gap. (a) Band structure of the La–Bi2201 sample with a doping level ofP=0.055 measured along the nodal direction at different temperatures. The data have been divided by the corresponding Fermi distribution functions to highlight the energy gap and the features above the Fermi level. (b) Original EDCs at the underlying Fermi momentum at different temperatures. (c) Corresponding EDCs after being divided by the Fermi distribution functions. (d) Symmetrized EDCs obtained fromb. Sample ageing has been checked by cycling temperature and the data are reproducible during the process. Figure 4 shows the temperature evolution of the band structure and the nodal gap in a typical La–Bi2201 sample with a doping level of 0.055. The measured data are divided by the Fermi distribution function ( Fig. 4a ) to visually inspect the energy gap as well as the possible features above the Fermi level. There is clearly a spectral weight suppression near the Fermi level for all the temperatures we have covered. This indicates that the nodal gap persists in the entire temperature range up to 300 K, close to the temperature of the possible pseudogap as determined by the NMR meausrements [6] . From the original EDCs on the underlying Fermi surface along the nodal direction ( Fig. 4b ), one can see that with increasing temperature, the coherence peak gets weaker and becomes indiscernible above 150 K, whereas the high-energy hump shows a slight change with temperature. The corresponding EDCs after dividing out the Fermi distribution function ( Fig. 4c ) exhibit a dip near the Fermi level, which together with the spectral distribution in the original data ( Fig. 4a ) indicate that the gap below and above the Fermi level is nearly symmetric. This justifies the procedure in symmetrizing EDCs to extract the energy gap in the paper. Figure 4d shows symmetrized EDCs on the underlying Fermi surface along the nodal direction; one can also see the persistence of the nodal gap till high temperatures. We do not show EDCs above 150 K in Fig. 4b–d because the disappearance of the coherence peak at high temperatures makes it difficult to quantitatively determine the gap size. Figure 4: Temperature dependence of the nodal gap. ( a ) Band structure of the La–Bi2201 sample with a doping level of P =0.055 measured along the nodal direction at different temperatures. The data have been divided by the corresponding Fermi distribution functions to highlight the energy gap and the features above the Fermi level. ( b ) Original EDCs at the underlying Fermi momentum at different temperatures. ( c ) Corresponding EDCs after being divided by the Fermi distribution functions. ( d ) Symmetrized EDCs obtained from b . Sample ageing has been checked by cycling temperature and the data are reproducible during the process. Full size image Momentum dependence of gap To investigate the momentum dependence of the energy gap in the lightly doped La–Bi2201, we have measured various momentum cuts along the underlying Fermi surface, picked up the EDCs along the underlying Fermi surface like in Fig. 2e,g,i,k , and extracted the gap size from the peak position of the symmetrized EDCs like in Fig. 2f,h,j,l . The obtained gap size as a function of momentum is shown in Fig. 5a–e for the La–Bi2201 samples with doping levels at 0.04, 0.055, 0.07, 0.08 and 0.10, respectively. It is clear that the gap is anisotropic and increases when the momentum moves from the nodal to the antinodal regions. For comparison, we also plotted an offset d -wave-like gap form Δ=Δ 0 cos(2Φ)+Δ N with Δ N representing the nodal gap (solid dashed lines in Fig. 5a–d ) and one can see that the measured data basically follow such a simple form in the samples with doping P =0.04–0.08. This is consistent with the previous report that d -wave-like gap is observed in the parent compound Ca 2 CuO 2 Cl 2 (ref. 19 ), insulating Bi 2 Sr 2 CaCu 2 O 8+ δ (Bi2212) (ref. 20 ), heavily underdoped Bi2212 (ref. 21 ) and underdoped (La 2– x Sr x )CuO 4 (ref. 22 ). The presence of the nodal gap indicates that the underlying Fermi surface is fully gapped for these samples. At the critical doping P ~0.10 where SC emerges, it shows zero gap near the nodal region, which is consistent with the ‘Fermi arc’ picture in the pseudogap state of other copper-oxide superconductors [12] , [13] . 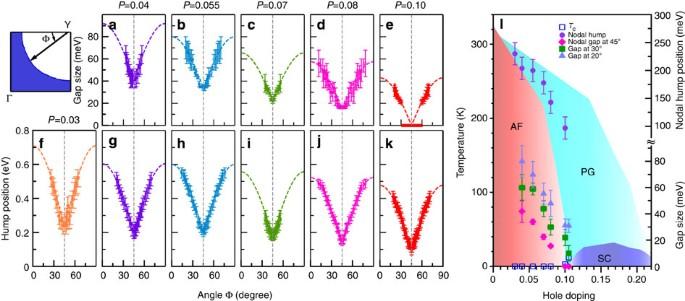Figure 5: Momentum dependence of the energy gap and its evolution with doping. The data were taken at a temperature of 20 K in lightly doped La–Bi2201 samples. (a–e) show the momentum dependence of the energy gap with different doping levelsPof 0.04 (a), 0.055 (b), 0.07 (c), 0.08 (d) and 0.10 (e). The Φ angle is defined in the top-left inset with Φ=45° corresponding to the nodal direction. The gaps are symmetrized with respect to the nodal direction for better visualization (empty circles). The dashed lines depict the offsetd-wave form Δ=Δ0cos(2Φ)+ΔNwith the offset ΔNcorresponding to the nodal gap. Error bars ina–ereflect the maximum deviation of the fitting process. (f–k) Momentum evolution of the hump for La–Bi2201 samples with different doping levelsPof 0.03 (f), 0.04 (g), 0.055 (h), 0.07 (i), 0.08 (j) and 0.10 (k). The dashed lines represent a form ofPh=Ph0cos(2Φ)+PhNwithPhNrepresenting the hump position along the nodal direction. Error bars inf–kaccount for the uncertainty in the determination of the high-energy hump position. (l) Phase diagram of La–Bi2201 system. It shows the 3D antiferromagnetic region defined byTN, superconducting region defined byTcand the pseudogap region defined byT*.TNandT* are reproduced from the previous NMR measurements6.Tcis determined from our magnetization and resistivity measurements. The doping dependence of the nodal gap size (pink diamond) and the nodal hump position (violet circles) is plotted. The energy gap away from the nodal direction, with Φ=30° (green solid squares) and 20° (blue solid triangles) is also plotted. We note that atP~0.10, the nodal gap goes to zero, the 3D AF vanishes (TNgoes to zero) and SC starts to emerge. The error bars for the gap and the hump are defined in the same way as ina–eandf–k, respectively. Figure 5f–k shows the position of the high-energy hump as a function of momentum for the La–Bi2201 samples at different doping levels. The broad hump structure also exhibits anisotropic momentum dependence with its position following a form P h = P h0 cos(2Φ)+ P hN with P hN representing the hump position along the nodal direction ( Fig. 5f–k ). The hump structure exhibits a minimum in binding energy along the nodal direction and its position decreases with the increase of doping levels. The similar momentum dependence of both the energy gap and the hump, and their similar doping dependence, suggest that they are intimately related, as will be discussed more below. Figure 5l illustrates the evolution of the energy gap and its relation with the 3D AF and SC [6] . At a critical doping level of P ~0.10, the nodal gap approaches zero, the 3D AF vanishes, and SC starts to emerge. Figure 5: Momentum dependence of the energy gap and its evolution with doping. The data were taken at a temperature of 20 K in lightly doped La–Bi2201 samples. ( a – e ) show the momentum dependence of the energy gap with different doping levels P of 0.04 ( a ), 0.055 ( b ), 0.07 ( c ), 0.08 ( d ) and 0.10 ( e ). The Φ angle is defined in the top-left inset with Φ=45° corresponding to the nodal direction. The gaps are symmetrized with respect to the nodal direction for better visualization (empty circles). The dashed lines depict the offset d -wave form Δ=Δ 0 cos(2Φ)+Δ N with the offset Δ N corresponding to the nodal gap. Error bars in a – e reflect the maximum deviation of the fitting process. ( f – k ) Momentum evolution of the hump for La–Bi2201 samples with different doping levels P of 0.03 ( f ), 0.04 ( g ), 0.055 ( h ), 0.07 ( i ), 0.08 ( j ) and 0.10 ( k ). The dashed lines represent a form of P h = P h0 cos(2Φ)+ P h N with P h N representing the hump position along the nodal direction. Error bars in f – k account for the uncertainty in the determination of the high-energy hump position. ( l ) Phase diagram of La–Bi2201 system. It shows the 3D antiferromagnetic region defined by T N , superconducting region defined by T c and the pseudogap region defined by T *. T N and T * are reproduced from the previous NMR measurements [6] . T c is determined from our magnetization and resistivity measurements. The doping dependence of the nodal gap size (pink diamond) and the nodal hump position (violet circles) is plotted. The energy gap away from the nodal direction, with Φ=30° (green solid squares) and 20° (blue solid triangles) is also plotted. We note that at P ~0.10, the nodal gap goes to zero, the 3D AF vanishes ( T N goes to zero) and SC starts to emerge. The error bars for the gap and the hump are defined in the same way as in a – e and f – k , respectively. Full size image Our observation of the nodal gap, and hence a fully gapped underlying Fermi surface in the lightly doped La–Bi2201 samples ( P =0−0.10) indicates that they have an insulating ground state. This is in a good correspondence to the transport measurements where the insulating behaviour is observed until P =0.08 in the resistivity–temperature dependence ( Fig. 1a ). Previous optical measurements also indicated a gap opening with the transition from metal to insulator near a doping of P ~0.10 in La–Bi2201 (ref. 23 ). The temperature dependence of the resistivity fits well with the model of 2D variable-range hopping of localized charges ( Fig. 1c ). For lightly doped samples, there is a semiconducting or insulating behaviour observed in the resistivity–temperature dependence [24] , [25] , but it is unclear whether it is a character of an intrinsic band insulator or a charge localization effect. Our results favour the latter. Our work clearly indicates that there is a true gap opening or complete loss of spectral weight at the Fermi level along the entire underlying Fermi surface so that the lightly doped samples are insulators. As shown by Gros et al. [10] , the high-intensity contour in the spectral weight distribution corresponds to the underlying Fermi surface only when the gap is small. As we focus mainly on the nodal region where the gap is relatively small, the maximal intensity contour is close to the underlying Fermi surface and the gap we have observed represents the one that opens up on top of the Fermi surface because of correlation. We note that, although the nodal gap has been reported before in a number of underdoped cuprates [21] , [22] , [26] , our observations are different in an important aspect. It was reported that a nodal gap is observed in the underdoped but superconducting Bi2212 above T c [21] , although there were different reports that no nodal gap is present even in a highly underdoped insulating Bi2212 sample [20] , [27] . For the underdoped Bi2212 sample with a T c near 34 K, which was reported to exhibit a nodal energy gap, its resistivity–temperature dependence shows a good metallic behaviour over an entire temperature range [28] . In (La 2– x Sr x )CuO 4 system, a nodal gap was reported at a doping level of 0.08 with a T c at 20 K [22] , although transport measurements also indicate that it is already a good metal over a whole temperature range [24] , [25] . These results suggest that the nodal gap, the pseudogap and the superconducting gap can occur at the same doping level [21] , [22] . In our case of La–Bi2201, it is clear that the nodal gap is competing with the superconducting gap: SC starts to emerge only after the nodal gap disappears. We note that the super-high-resolution ARPES measurements enable us to observe clear coherence peaks even in the heavily underdoped samples, thus making it possible to get a precise determination of the energy gap. Also, for many samples investigated in the present study, they have the same composition; the doping is slightly tuned by varying the oxygen content during the annealing process. The existence of the nodal gap in the lightly doped La–Bi2201 samples ( P <0.10), together with other characteristics like the peculiar doping, momentum and temperature dependence, puts constraints on its underlying origin of formation. The coincidence of the nodal gap disappearance and the vanishing of the 3D AF near P ~0.10 indicates that long-range AF is closely related to the electronic structure evolution across the insulator–superconductor transition. It is natural to ask whether the static antiferromagnetic order alone can give rise to the energy gap formation in the lightly doped region. As it is well known, the presence of static antiferromagnetic order can double the unit cell in real space and reduce the Brillouin zone in the reciprocal space by half. This would cause band folding that will make the initial ‘large Fermi surface’ and folded Fermi surface cross somewhere in between the nodal and antinodal regions. This is most clearly demonstrated in the electron-doped cuprates [29] . This picture alone cannot explain the gap formation near the nodal region, it cannot explain the anisotropic d -wave-like gap form either. Very recently, it was pointed out by theoretical calculations that the nodal d -wave spectrum is robust against strongly fluctuating competing order-like antiferromagnetic correlation. However, when the antiferromagnetic correlation is strong and the phase has spatial inhomogeneity, a nodal gap can be developed that grows with the antiferromagnetic magnitude [30] . This picture may be able to account for the nodal gap opening in the lightly doped region. However, the result is obtained in a weak coupling approach and it shows a strong temperature dependence that is different from what we have observed. Another possibility to consider is whether the energy gap can be induced by disorder because it can give rise to localization, which leads to insulating behaviours. In doped semiconductors, which show variable-range hopping, there is a long-range Coulomb effect that can depress the density of states near the Fermi energy forming the so-called ‘Coulomb gap’ [31] , [32] . As our La–Bi2201 samples ( P <0.10) are insulating at low temperature with their transport property consistent with the variable-range hopping picture ( Fig. 1c ), this effect may be present. The disorder scenario can in principle account for our observation of the nodal gap; it was proposed to explain the normal-state antinodal gap before [18] . In this picture, it is also possible to explain the nodal gap increase with decreasing doping because the screening of the Coulomb interaction gets weaker. However, it is unclear whether such an interaction effect can produce a d -wave-like anisotropic energy gap and why the disappearance of the nodal gap coincides with the vanishing of the long-range AF. The presence of the high-energy hump does not have a natural explanation from the disorder effect either. One may invoke strong electron correlation that can generate a hump structure as the incoherent background, which lies below the coherent states near the Fermi level [33] . It has been recently shown theoretically that disorder can drive an insulator–superconductor transition at a critical disorder strength and produce a single particle gap [34] . These aspects bear similarities to our observations of the nodal energy gap and an insulator–superconductor transition near P ~0.10. However, it predicts that the nodal gap exists for both the insulating region and the superconducting region, which is inconsistent with our observation that the nodal gap exists only in the insulating samples. It is known that in the heavily underdoped regime, charge ordering like the diagonal stripe may be formed, as observed in La 2– x Sr x CuO 4 (LSCO) system [35] , [36] as well as Bi 2– x Sr 2+ x CuO 6+ y (Bi2201) system [37] . It was suggested that the diagonal stripe can be understood in terms of the conventional spin-density wave (SDW) picture, originating from nesting of nodal states [38] . Such SDW is expected to open a gap and localize the nodal states that prevent the SC from occurring. When the diagonal SDW vanishes, the gap closes, the nodal states are recovered and SC emerges. These appear to agree with our results that the nodal energy gap approaches zero when the SC emerges. However, from the diagonal stripe scenario, it is not clear why the disappearance of the nodal gap coincides with the vanishing of the long-range AF. It is also unclear why the gap takes an anisotropic d -wave-like gap form, as the nesting order would open a gap only on the nested segments of the Fermi surface [39] . The systematic doping evolution of the photoemission spectra, that is, the emergence of the coherence peak with a slight doping, the coexistence of the coherence peak with a broad hump and their coordinated evolution with doping ( Figs 3h and 5 ), is reminiscent of observations in other copper-oxide compounds [15] , [16] , some one-dimensional materials [40] and bilayer manganite La 1.2 Sr 1.8 Mn 2 O 7 (ref. 41 ). These behaviours can be reasonably explained by the formation of small polarons [16] , [40] , [42] , [43] with electrons dressed by spin excitations or lattice vibrations. This polaron picture can explain the lineshape of the photoemission spectra [16] , [40] , [42] , [43] . However, it does not provide a satisfactory explanation for the energy gap because, in a simple polaron picture, the primary coherence peak is expected to stay at the Fermi level [40] . Theoretical calculations [44] , [45] have shown that AF can enhance the effective electron–phonon interaction that makes it possible for the formation of the self-trapped polarons. Once the self-trapped polaron is formed, the spectral weight of the quasiparticle at the Fermi level is reduced to zero [45] . In addition, there are several peaks appearing at higher binding energies, as the motion of the charge is strongly coupled with the creation of spin-wave excitations and phonons. Therefore, in the extremely low doping region (like P =0.03 and below) with a strong antiferromagnetic order, the effective electron–phonon interaction is very strong, those peaks appeared at a rather high binding energy without spectral weight at the Fermi level, leading to the appearance of a large gap. With increasing doping (like P =0.04–0.08), the peaks would move towards the Fermi level, accompanied by a decrease of the gap size. When the effective electron–phonon interaction reduces below a critical value, the gap approaches zero and the electron–phonon interaction is simply to renormalize the quasiparticle mass with a finite spectral weight at the Fermi level. Our observation of the simultaneous disappearance of the AF and the nodal gap (or lack of spectral weight at the Fermi level) seems to agree quite well with this picture. One important prediction of the theories [45] , [46] is that the momentum dependence of the peaks at higher binding energies follows the same energy dispersion of the quasiparticles without any electron–phonon interaction. Thus, the d -wave-like momentum dependence of the ARPES spectra shown in Fig. 5 can be naturally understood. We also note that Fig. 5a–e shows a rigid energy shift along almost the entire Fermi surface. Any mechanism for the formation of the nodal gap should not modify the Fermi surface and the polaron picture is a natural candidate for this effect. Although the polaron scenario seems quite plausible for our observations, we still need a more quantitative explanation of the spectral lineshape for the insulating regime. To this end, a more comprehensive calculation may be necessary to include both the electron–phonon interaction and long-range Coulomb effect together with the AF. One important question to ask is the relationship between the energy gap observed in the insulating samples ( x =0–0.08) and the pseudogap observed in the underdoped superconducting region ( x =0.10–0.15). In Fig. 5l , for several given momenta, we plotted the energy gap observed in the insulating region ( x =0–0.08) and the pseudogap observed in the underdoped superconducting region ( x =0.10–0.105). The region with the insulating gap smoothly evolves into the pseudogap region without an abrupt change. In conjunction with the d -wave-like gap form, the decrease of the nodal gap as doping increases from 0.04 to 0.10 also reduces the gap value at the antinodal region to about 40 meV, which is close to the maximum pseudogap value observed for the superconducting phase [20] . This is the first experimental evidence that has been presented about the continuous increase of the pseudogap at the antinodal region as the system crosses from the superconducting phase to the insulating antiferromagnetic phase. Our result of the d -wave-like gap form is qualitatively consistent with the idea that the d -wave-like spin singlet pairing already exists in the insulating parent compound and lightly doped samples [47] . It is theoretically shown that, even if there is a long-range antiferromagnetic order, energy dispersion still has the d -wave-like form along the Fermi surface [48] . However, due to the presence of the antiferromagnetic phase, the electron–phonon interaction is greatly enhanced to create polarons and needs to be considered to account for the spectral lineshape and the nodal gaps we have observed. As the antiferromagnetic fluctuation and electron–phonon coupling are present well into the higher doping region in spite of their reduced strength [43] , one may expect they also have an important role in dictating the electronic structure and properties in higher doping regions. In conclusion, we have observed a clear insulator–superconductor transition in the La–Bi2201 system near the doping level of ~0.10. The results reveal an intimate relation between SC and AF, that is, SC emerges at the critical doping level where 3D antiferromagnetic order vanishes and the nodal gap disappears. These observations are qualitatively consistent with the formation of self-trapped polarons in the lightly doped samples. They indicate that antiferromagnetic correlation and the strong electron–phonon interaction are important to understand the electronic structure and anomalous physical properties of cuprates, at least in the underdoped region. Sample preparation and estimation of doping levels The Bi 2 Sr 2– x La x CuO 6+ δ (La–Bi2201) single crystals were grown by the travelling solvent floating zone method [49] . We obtained various dopings by changing the La concentration and postannealing under different temperatures and atmospheres: the sample with the hole concentration P =0.03 has a composition of x =1.02, whereas all the other samples with hole concentrations of 0.04, 0.055, 0.07, 0.08, 0.10 and 0.105 have the same composition with x =0.84 but annealed under different conditions. The La–Bi2201 samples are characterized by different measurements, including magnetization measurements, the temperature dependence of the resistivity and the Hall coefficient measurements. The doping level p in La–Bi2201 is determined by a couple of factors including La-content, oxygen content, inter-exchange between Bi and Sr and so on. Because of these complications, the precise determination of the doping level p is not straightforward but was estimated in the literature from combined transport measurements like resistivity, Hall coefficient and the thermoelectric power. In our present work, we followed a similar procedure to estimate the doping levels by comparing our data with those in the literature that already provided a good correspondence between the doping concentration, T c and resistivity–temperature dependence [50] . Note that we used similar single-crystal growth procedures as used by the other groups [6] , [50] so the doping levels between the samples are presumably comparable. The La–Bi2201 samples with hole concentrations p of 0.03, 0.04, 0.055, 0.07 and 0.08 are non-superconducting. The P =0.10 sample is superconducting with a transition temperature T c ~3 K, near the border of non-superconductor to superconductor transition. The P =0.105 sample shows a T c of 12 K. High-resolution ARPES measurements The ARPES measurements were carried out on our vacuum ultraviolet laser-based angle-resolved photoemission system with advantages of high photon flux, enhanced bulk sensitivity and super-high-energy and momentum resolution [51] . The photon energy is 6.994 eV with a bandwidth of 0.26 meV. We set the energy resolution of the electron energy analyser (Scienta R4000) at 1.5 meV, giving rise to an overall instrumental energy resolution of 1.52 meV. The angular resolution is ~0.3°, corresponding to a momentum resolution of ~0.004 Å −1 . The samples were cleaved in situ and measured under ultrahigh vacuum better than 4 × 10 −11 Torr. How to cite this article: Peng, Y. et al. Disappearance of nodal gap across the insulator–superconductor transition in a copper-oxide superconductor. Nat. Commun. 4:2459 doi: 10.1038/ncomms3459 (2013).